A principal component meta-analysis on multiple anthropometric traits identifies novel loci for body shape Large consortia have revealed hundreds of genetic loci associated with anthropometric traits, one trait at a time. We examined whether genetic variants affect body shape as a composite phenotype that is represented by a combination of anthropometric traits. We developed an approach that calculates averaged PCs (AvPCs) representing body shape derived from six anthropometric traits (body mass index, height, weight, waist and hip circumference, waist-to-hip ratio). The first four AvPCs explain >99% of the variability, are heritable, and associate with cardiometabolic outcomes. We performed genome-wide association analyses for each body shape composite phenotype across 65 studies and meta-analysed summary statistics. We identify six novel loci: LEMD2 and CD47 for AvPC1, RPS6KA5 / C14orf159 and GANAB for AvPC3, and ARL15 and ANP32 for AvPC4. Our findings highlight the value of using multiple traits to define complex phenotypes for discovery, which are not captured by single-trait analyses, and may shed light onto new pathways. Large-scale meta-analyses of genome-wide association studies (GWAS) have identified numerous loci for anthropometric traits, including more than 600 loci for height [1] , [2] , [3] and over 160 loci for obesity-related outcomes, predominantly for commonly available traits such as body mass index (BMI) [2] and waist-to-hip ratio (WHR) [4] , [5] , but also for body fat percentage [6] , childhood obesity [7] and extreme and early onset obesity [7] , [8] , [9] . While GWAS-meta-analyses have successfully revealed new loci, so far, all these studies have focused on one single anthropometric trait at a time and may not adequately capture differences in body shape between individuals who are similar in one trait but different in others. For example, two individuals may have the same BMI, but their WHR and/or height can differ substantially, so that each has a different body shape, which may translate into differences in disease risk [10] , [11] . Several loci identified from previous single-trait GWAS on BMI, BMI-adjusted WHR (WHRadjBMI) and height are associated with more than one anthropometric trait [1] , [2] , [4] , [12] . For example, the loci near MC4R and near POMC/ADCY3 are each associated with BMI and height. However, the BMI-increasing allele of the near- MC4R locus is associated with increased height, whereas the BMI-increasing allele of the near- POMC/ADCY3 locus is associated with reduced height [1] , [2] . Thus, these loci are likely each associated with a more comprehensive body shape phenotype that is not captured by current GWAS that only consider anthropometric traits individually. In recent years, several approaches have been developed to examine whether single-nucleotide polymorphisms (SNPs) influence multiple correlated traits associated with disease [13] , [14] . However, most approaches test phenotypes separately and are thus subject to multiple testing penalties that ultimately reduce the statistical power to detect genotype–phenotype relationships among correlated traits. One way forward is to apply a dimension reduction method to the traits of interest, such as principal component analysis (PCA) that combines multiple correlated traits into a set of uncorrelated outcomes principal components(principal components (PCs)) [15] , [16] . This method is very appealing to capture a composite phenotype, such as body shape. To date, no large-scale GWAS meta-analyses have been reported that aim to identify genetic loci associated with body shape based on simultaneous analysis of multiple anthropometric traits using PCA methods. Therefore, the purpose of our study was twofold. First, we aimed to capture body shape in its multi-dimensional structure using PCs from several commonly available anthropometric traits. To allow the meta-analysis of summary statistics across a large number of cohorts, we developed an approach that calculates averaged PCs (AvPCs) that robustly represent body shape across a wide range of studies. Second, using this approach, we aimed to identify genetic loci associated with body shape based on the AvPCs in 65 studies of the GIANT Consortium, including >170,000 individuals. Defining composite phenotypes of body shape As basis for our analysis of body shape we used six anthropometric traits: BMI, WHR, height, weight, hip and waist circumference. 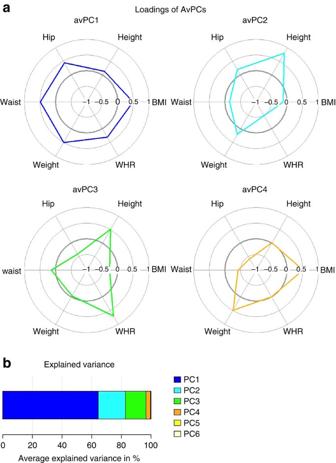Figure 1: Loadings and explained variance of AvPCs for body shape. (a) Loadings of AvPCs, and (b) explained variance of AvPCs for body shape. First, we performed separate PCA in a subset of 20 large population-based studies (up to 82,355 individuals, Supplementary Table 1 ) and compared the loadings of the anthropometric traits in each PC between studies. Visual inspection of PCA loadings showed high concordance across studies ( Supplementary Fig. 1 ) and between men and women. Between-study variation in variance explained by the PCs was small ( Supplementary Fig. 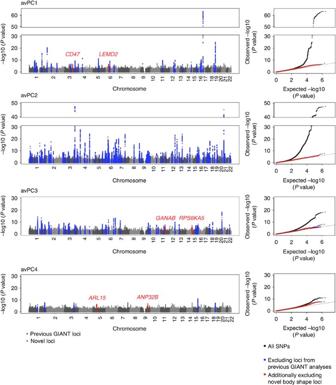Figure 2: Manhattan and QQ-plots of association results on AvPCs of body shape. Pvalues of the first stage meta-analysis are given in the Manhattan and QQ-plots. All genome-wide significant loci are highlighted. 1 , Supplementary Table 2 ). On average, the first four PCs explained more than 99% of the variance ( Fig. 1 , Supplementary Table 2 ), and were therefore pursued as body shape outcomes for our gene-discovery effort. Given the across-study stability of PCs, we derived average loadings that were calculated as weighted means of loadings from all 20 population-based studies that were analysed in this step. We used these average loadings to calculate average principal components (AvPCs) as targets in each of the GWAS included in the first and second stage. In other words, the phenotypes used for genome-wide association were constructed in a consistent way across studies, such that the summary statistics could be meta-analysed. Figure 1: Loadings and explained variance of AvPCs for body shape. ( a ) Loadings of AvPCs, and ( b ) explained variance of AvPCs for body shape. Full size image Each AvPC represents a specific composition of the six anthropometric traits and thus captures a specific aspect of body shape ( Fig. 1 ). The first AvPC, which explains on average 64.4% of the variation in all traits, shows high loadings for all traits, except for height. The loadings are in the same direction; meaning that the AvPC captures inter-individual variation in either increased or decreased BMI, weight, WHR, hip and waist circumference. Therefore, variation in this PC seems to predominantly capture overall adiposity. The second AvPC, which explains 18.5% of the variation, is characterized by particularly high but opposite loadings on height and WHR. In other words, AvPC2 captures variation in a composite phenotype that represents tall individuals with a small WHR or, vice versa, short individuals with a large WHR. The third AvPC, explaining 13.8% of the variation, also shows predominantly high loadings on height and WHR but in the same direction, with an opposite loading of nearly the same size on hip circumference. Given these loadings, AvPC3 discriminates mainly between tall individuals with a high WHR resulting from a smaller hip circumference on one extreme and short individuals with low WHR, and a larger hip circumference on the other extreme. The fourth AvPC explains on average 3% and is harder to interpret. It displays high loadings on BMI and body weight, and opposite loadings of a similar size on hip and waist circumference. These could be interpreted as a phenotype ranging between high BMI and weight, with relatively small hip and waist circumference on the one hand and low BMI and weight but large waist and hip circumference on the other hand. Consistent with the individual anthropometric traits, the four AvPCs that describe body shape are also heritable. Using data from four isolate populations ( n =4,000), we estimated that AvPC2 has the highest heritability (75–80%), consistent with the fact that height is the main contributing trait to this AvPC with a strong genetic component [1] . The heritability of AvPC1 (35–50%), AvPC3 (50–75%) and AvPC4 (25–50%) were moderately high and similar to the heritability for individual anthropometric traits [17] ( Supplementary Fig. 2 ). From a clinical perspective, each of the four AvPCs exhibit known correlations with cardio-metabolic traits ( Supplementary Fig. 3 ), including diastolic blood pressure, systolic blood pressure, total cholesterol, low-density lipoprotein cholesterol, high-density lipoprotein cholesterol and total triglycerides levels. 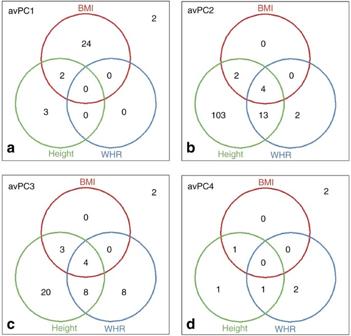Figure 3: Number of loci associated with AvPCs and known from previous GIANT analyses on BMI, WHR or height. (a–d) corresponds to each AvgPC respectively. The Venn diagrams specify for each AvPC how many significantly associated loci (promisingPvalue in the first stage meta analysis (<5 × 10−6) and genome wide significant in first and second stage combined analysis (<5 × 10−8)) are known from previous GIANT analysis on BMI, height or WHR. In the upper right corner of each plot the number of loci is given that are not known from previous GIANT analyses. Genomic discovery of body shape composite phenotypes We performed a two-staged meta-analysis to identify genetic loci that are associated with the four AvPCs ( Supplementary Table 3 , Supplementary Table 4 ). In the first stage, a meta-analysis of 43 studies with imputed genome-wide SNP data including more than 133,000 individuals identified SNPs in 385 loci across the four AvPCs (56 loci for AvPC1, 205 for AvPC2, 89 for AvPC3 and 35 for AvPC4) that showed promising association ( P value<5 × 10 −6 ) for at least one of the four AvPCs ( Fig. 2 , Supplementary Fig. 4 ). Lead SNPs (and proxies; see ‘Methods’ section) of each locus were taken forward for validation in a second stage, including data from more than 39,900 individuals from 22 studies of which 12 studies had genotypes from the Illumina CardioMetabochip and 10 studies had imputed genome-wide SNP data. In the combined analyses, consisting of the first and second stage studies, the association of 207 of the 385 loci reached genome-wide significance ( P value <5 × 10 −8 ) (31 for AvPC1, 124 for AvPC2, 45 for AvPC3 and 7 for AvPC4; Fig. 2 , Fig. 3 , Supplementary Fig. 4 , Supplementary Table 6 ), of which 16 loci were identified for two AvPCs and one showed significant association with three AvPCs ( Supplementary Fig. 7 , Supplementary Table 5 ) resulting in a total of 189 loci with association to at least one AvPC. To determine whether the loci we identified were independent of the loci previously found for BMI, WHRadjBMI and height, we performed conditional analyses on SNPs reported in previous GIANT-GWAS publications on BMI, WHRadjBMI and height [1] , [2] , [4] , [5] , [18] , [19] . A locus was considered independent of reported findings if the P value in the analyses conditioned on all previously identified loci remained suggestive ( P value <5 × 10 −6 ). In total, 183 loci had already been established for BMI, WHRadjBMI or height ( Fig. 3 , Supplementary Fig. 7 ), whereas six loci had not previously been identified for association with conventional anthropometric traits; two for AvPC1, two for AvPC3 and two for AvPC4 ( Table 1 , local association plots given in Supplementary Fig. 5 ). For these six novel loci, the results of the lead SNPs were checked in previously performed GWAS meta-analyses on anthropometric and cardio-metabolic traits ( Supplementary Table 7 ). Figure 2: Manhattan and QQ-plots of association results on AvPCs of body shape. P values of the first stage meta-analysis are given in the Manhattan and QQ-plots. All genome-wide significant loci are highlighted. Full size image Figure 3: Number of loci associated with AvPCs and known from previous GIANT analyses on BMI, WHR or height. ( a–d ) corresponds to each AvgPC respectively. The Venn diagrams specify for each AvPC how many significantly associated loci (promising P value in the first stage meta analysis (<5 × 10 −6 ) and genome wide significant in first and second stage combined analysis (<5 × 10 −8 )) are known from previous GIANT analysis on BMI, height or WHR. In the upper right corner of each plot the number of loci is given that are not known from previous GIANT analyses. Full size image Table 1 Association results for novel loci with avPC of body shape. Full size table Results for AvPC1 For AvPC1, we identified 31 genome-wide significant loci, of which two were novel (upstream of LEMD2 and CD47 ). Of the 29 previously established loci, 24 have been associated with BMI only [18] , 3 with height only [1] , [3] , while two loci have been reported for associations with both BMI and height [3] , [18] ( Fig. 3a ). While both novel loci showed some evidence of association with BMI in the latest GIANT–GWAS ( n >339,000; P <7.2 × 10 −3 ; Table 1 ), they did not reach genome-wide significance. The lead SNP (rs943466) 7 kb upstream of LEMD2 has been reported to be associated with expression of LEMD2 in liver ( P =1.66 × 10 −9 ) [20] , [21] . Another variant in LEMD2 ( rs2296743 at 8 kb from our lead SNP rs943466; r 2 =0.2, D′=1.0) was previously reported for its promising association ( P value=8 × 10 −6 ) with energy intake at dinner in a small GWAS of 815 Hispanic children [22] . The lead SNP (rs7640424) for the second novel locus was located in an enhancer region 10 kb upstream of CD47 (refs 23 , 24 ), which encodes a membrane protein that might be involved in signal transduction and membrane transport [25] . No genome-wide significant associations have been reported for the lead SNP or other SNPs in the CD47 gene before [23] , [24] , [25] . However, a recent study revealed a link to diet-induced obesity in mice and suggests CD47 as a potential drug-target to combat obesity and metabolic complications [26] , [27] . Results for AvPC2 For AvPC2, we identified no novel loci. Almost all ( n =122) of the 124 loci associated with AvPC2 had previously been identified for height [1] ( Fig. 3b ), which is consistent with AvPC2’s high loadings on height and opposite loadings on WHR. Of these 122 loci, 103 were reported for association to height only, whereas of the 19 remaining loci, 4 were previously associated with height, BMI and WHRadjBMI, 2 loci were reported for height and BMI and 13 loci overlapped with height and WHR. The two AvPC2 loci that did not associate with height were previously identified for WHRadjBMI [19] . Results for AvPC3 We identified 45 loci that reached genome-wide significance for AvPC3, of which 2 were novel. Consistent with the loadings of AvPC3, 43 of the associated loci had been reported before for height [1] or WHR [4] , [19] ( Fig. 3c ). The lead SNP of the first novel locus rs7492628, upstream of the genes RPS6KA5 (>20 kb) and C14orf159 (>30 kb), failed to reach genome-wide significance in previous WHRadjBMI GWAS ( P value=9.3 × 10 −8 ) and was nominally associated with extreme obesity risk ( P value=7.26 × 10 −5 ) [28] . The lead SNP of the other novel locus, GANAB, rs7949030, showed some evidence of association with WHRadjBMI in the latest GIANT GWAS ( P value=3.3 × 10 −6 ) and was reported to be an eQTL for several other genes [21] : In monocytes, regulation of MIR3654 , EEF1G , EML3 , BSCL2 , HNRNPUL2-BSCL2 , LRRN4CL was found [29] , [30] , [31] . BSCL2 is of interest, as it is a known candidate gene for the most severe lipodystrophy phenotype [32] . In blood rs7949030 was found to be an eQTL of HNRNPUL2-BSCL2 , AHNAK , LRRN4CL and INTS5 (refs 33 , 34 ), while in skin and adipocytes it was found as an eQTL for EML3 (refs 30 , 31 , 35 ). Results for AvPC4 Seven loci were identified for AvPC4, of which five had been previously reported; one for BMI and height, one for WHR and height, one for height only and two for WHR only [1] , [3] , [4] , [36] ( Fig. 3 ). The lead SNPs of the two novel loci identified with AvPC4 were both intronic, in ARL15 and ANP32 . The allele associated with increased AvPC4 of the lead SNP (rs4865796) in ARL15 was moderately associated with higher BMI ( P value=1.6 × 10 −4 ), increased adiponectin levels ( P value=4.2 × 10 −6 ADIPOGEN [37] ) and decreased risk of diabetes ( P value=1.8 × 10 −5 , DIAGRAM [38] ). This SNP was associated with fasting insulin (rs4865796, P =2.1 × 10 −8 and 2.2 × 10 −12 after adjustment for BMI [39] ). Other nearby SNPs in high linkage disequilbrium (LD), have previously been reported for associations with BMI-adjusted adiponectin levels (rs6450176/rs4311394, r 2 =0.087, D′=0.87 (refs 37 , 40 )), high density lipoprotein C (HDL-C) levels (rs6450176 (refs 41 , 42 )) and risk of type 2 diabetes (rs702634, r 2 =1.0, D′=1.0 (ref. 38 )). A duplication in ARL15 , tagged by rs16992296) was previously found to be associated with increased risk of childhood obesity in European and African Americans [43] . However, this duplication is independent of the association we found for rs4865796-ARL15 and AvPC4, which is in low LD ( r 2 EUR=0.065) with the duplication (represented by rs16992296), located 168 kb upstream. The lead SNP (rs7855432) of the second locus, ANP32B, was moderately associated with height ( P value=5.5 × 10 −6 ) [1] . A SNP in high LD (rs4743150 r 2 =0.95, D′= 1.0) was reported to be promisingly associated with coronary heart disease risk ( P value=5 × 10 −6 ) [44] . We developed a PCA-based approach to capture variation across multiple traits simultaneously in a uniform way across multiple studies. Resulting AvPCs are a robust cross-phenotype representation allowing their use in large-scale meta-analyses. We assessed this approach to capture body shape based on six individual anthropometric traits and identified six novel loci that were not identified before in much larger GWAS-meta-analyses for BMI, WHRadjBMI and height [1] , [2] , [4] . Our findings suggest that the body shape composite phenotype, assessed by AvPCs, represents information that is not fully captured by individual (anthropometric) traits. Application of this method to other related traits, for example, in immune disease, different types of cancer, cardiometabolic traits, or other correlated traits might comparably reveal new loci, and potentially new pathways, that have not been identified in single-trait GWAS. The AvPCs are combinations of different anthropometric traits and therefore capture more complex body shape phenotypes than the single traits. AvPC1, representing overall adiposity, and AvPC2, representing height with respect to WHR, are the most important contributors to body shape, explaining on average more than 80% of the variation. More specific body shape types were captured by AvPC3 and AvPC4 and were defined by impact of height and WHR (AvPC3) or BMI, waist and hip (AvPC4). Our initial analyses demonstrated that the loadings are stable across studies, study designs and between men and women. Moreover, we have shown that the AvPCs are heritable traits and correlated with cardiometabolic traits and risk factors. To further demonstrate the strength of this approach, we compared total variance explained of single traits and AvPCs by SNPs previously identified in single-trait GWAS (for BMI, WHRadjBMI, height [1] , [2] , [4] ). For example, the 97 loci that have been reported for association in the latest BMI single-trait GWAS (N ∼ 340,000) explain 8.7% of the variation in AvPC1, whereas they explained only 2.68% of the variation in BMI [2] . These data indicate that our PC-defined phenotype for overall body size (AvPC1) captures a more composite phenotype compared with BMI as a single-trait. Explaining more of the variance with the same genetic variants as previous single-trait studies in our composite phenotype shows promise to update and inform existing methods. So far, typical GWAS have tested for association of genetic variants with anthropometric traits, one trait at a time. We define ‘body shape’ as a composite of multiple traits defined by PCs. We first performed PC-analyses in representative population-based studies and averaged PC loadings across these studies (AvPCs). We subsequently use these AvPCs to calculate PCs in all participating studies. This approach ensures that PCs are calculated in a uniform manner across all studies, thus facilitating subsequent meta-analyses. This approach could be applied to capture genetic variation across related traits that is currently not captured by single-traits GWAS (for example, in the context of autoimmune disease, blood traits, lipid levels, different cancers and so on.). Consistent with published anthropometric traits [10] , [11] , [17] , the derived AvPCs are heritable and correlated with clinically relevant outcomes. We identified additional loci, despite a much smaller sample size compared with the latest single-trait GWAS analyses for BMI, height and WHRadjBMI [1] , [2] , [4] . This suggests that the AvPC method captures phenotype information that is not captured by single-trait analyses and associated loci may highlight biological pathways that are not revealed with single-trait associated loci only. Even though our approach has several advantages, it is not meant to replace single trait GWAS analyses. A number of loci that were identified in the latest single-trait GWAS were not identified in our body shape GWAS; that is, we identified 124 loci (or 14.2%) of the 837 loci recently reported in the GIANT single-trait meta-analyses ( Supplementary Fig. 6 ). This may be due to the fact that these recent single-trait GWAS meta-analyses were at least twice as large as the current body shape GWAS. However, even when we compare the number of identified loci in earlier GWAS meta-analyses, which are of similar size as the current body shape GWAS, we do not identify all previously reported loci for single traits. Perhaps this is most obvious with height (largely representative of AvPC2), where we only identified 91 (13.1%) of 697 loci identified for height. This is in part due to the fact that a conservative definition for linkage disequilibrium was applied ( r 2 >0.8), lack of power due to sample size for SNPs of modest effects, or perhaps the AvPCs introduces noise to purely single traits such as height. Consistent with this finding, we also observe that some single traits also explain more of the variance of body shape compared with AvPCs. Our comparison of the variance explained between previous single-traits meta-GWAS and our AvPCs support this evidence for overlapping associated variants. Since AvPC2 represents largely a single trait, height, with large height loadings we were unable to explain more of the variance. In fact we explained less of the variance, which is likely due to noise introduced using this composite AvPCs phenotype. This observation is also evident for variance in body shape explained by height compared with AvPC3 and AvPC4, but is in contrast to BMI, a complex trait comprised of multiple anthropometric measurements, which explains less variance in body shape compared with AvPC3 and AvPC4. It is important to emphasize our approach is most informative for complex traits such as BMI that are derived from a series of other traits. We believe that using PC space to define complex traits is useful for the detection of loci involved in multiple pathways that might go undetected in a single trait setting. We have developed a new strategy that applies a PCA approach in a meta-analysis setting to combine composite phenotypes in a harmonized way across multiple studies. We successfully applied this approach to anthropometric traits to capture body shape. The derived combined anthropometric traits (AvPCs) were shown to be heritable and correlated to cardio-metabolic traits. Large-scale GWAS meta-analyses of the AvPCs identified six new loci that were not identified by previous single-trait GWAS that were twice as large in samples size. This PCA approach could maximize gene discovery for other correlated traits, such as cancers, immune disease, hematologic traits and so on. and may identify genes that point towards shared physiological pathways. Study description In the first stage analyses, 43 studies participated (133,376 individuals) that had HapMap 2 imputed genome-wide data available. A subset of 20 studies with unrelated individuals was used for calculation of average loadings. Second stage analyses were performed in 10 studies (7,734 individuals) with genome-wide data that became available after the first stage and 12 studies (32,170 individuals) with Cardio-MetaboChip (by Illumina) data (number of included studies and individuals given in Supplementary Table 3 ). Details on study phenotypes, genotyping and imputation of each study are given in the Supplementary Tables 8 and 9 , respectively. Ethics statement All study participants gave written informed consent and ethic committees approved all studies. The ethic statement of each study is given in the study specific acknowledgements. Calculation of average loadings In 20 independent studies ( Supplementary Table 1 ) with unrelated participants PCAs were performed on six anthropometric traits (BMI, height, hip, waist, weight and WHR). Each study performed a PCA on the standardized residuals of the anthropometric traits adjusted for age and gender. The same analyses were done for men and women separately with residuals adjusted for age only. The result of the PCA in each study is a set of six PCs that are orthogonal linear combinations of the six anthropometric traits. In other words each PC is a weighted sum of the six transformed anthropometric traits and independent of the other PCs. The weights of each trait per PC are called loadings. Each study also calculated the explained variance per PC. The loadings and explained variances were comparable for all studies ( Supplementary Fig. 1 (1)). With the intention to create phenotypes that are identically constructed in all studies, the results of single study PCAs were used to deduce the average loadings. This approach is reasonable as the loadings of the study specific PCAs were comparable. With the use of the single study correlation matrices a combined average correlation matrix was derived (weighted sum divided by number of individuals). This average correlation matrix is then used as basis for a PCA. The loadings that result from this PCA are called average loadings ( Fig. 1a ) and Supplementary Table 2 ). This was performed for men, women and all individuals combined, however ultimately we used combined loadings for primary results reported in the manuscript. Sex specific results are reported in the Supplementary Material . The average loadings and explained variance were comparable to the study specific loadings and explained variances ( Supplementary Fig. 1 ). Heritability analyses Heritability of the avPCs was calculated within four population isolates, CROATIA-Vis ( n =909), CROATIA-Korcula ( n =842), CROATIA-Split ( n =499) and ORCADES ( n =866) using the ‘polygenic’ function of the GenABEL package for R [45] . Average principal components as body shape phenotype The average loadings were used in each study to calculate the AvPCs in a standardized way. Therefore, the average loadings were distributed together with an R-script ( http://www.r-project.org/ ) that calculated the AvPCs as linear combination of residuals of the study phenotypes with the use of the average loadings. This was done for men and women separately and additionally for combined in studies with relatedness structure. As the first four PCs explain on average more than 99% of the variance ( Fig. 1b ) we decided to limit all analyses to these four PCs. Stage 1 analyses GWAS on the first four AvPCs were calculated for men and women separately in studies of unrelated samples and combined for studies with related samples with an adjustment for study site when necessary. All studies of the first stage analyses used HapMap 2 imputed genome-wide data. GWAS results underwent extensive quality control and study-wise filtering (call rate >95%, P value (HWE)>10 −6 , imputation quality, minor allele count (MAC) >3). The meta analyses of GWAS results for the first four AvPCs we combined sex-stratified results for studies with unrelated individuals and unstratified GWAS results for studies with relatedness individuals. Meta analyses were performed with METAL [46] using fixed effects inverse variance-weighted method. Single study and the meta analysis P values were corrected by the genomic control inflation factor λ (meta analysis λ before correction: λ (PC1)=1.29, λ (PC2)= 1.407, λ (PC3)= 1.236, λ (PC4)= 1.136). Results were limited to SNPs that are in HapMap 2 and had results for more than 30,000 individuals. Heterogeneity analysis was performed with METAL. Each AvPC all SNPs with a promising P value ( P value<5 × 10 −6 ) were identified in combined analyses. To identify promising loci clustering (LD>0.01, distance <1,000 kb) with PLINK [47] based on HapMap 2 genotypes was performed. All leading SNPs per clump for AvPCs were taken forward to second stage analyses and named promising SNPs in this manuscript. Two SNPs that were promising for the first principal component had very low heterogeneity P values (rs10847678 ( P value(het)=8.8 × 10 −152 ), rs13296358 ( P value(het)=5.4 × 10 −67 )). For both SNPs the effect was driven only by a single study and no other SNP in high LD had a promising P value. Therefore, these two SNPs were removed from further analyses. Stage 2 Analyses As mentioned above for second stage analyses a mixture of studies with genome-wide SNP data and MetaboChip genotypes was available. Some of the leading SNPs of the first stage analyses were not genotyped on the MetaboChip. To increase the power for all promising SNPs of each AvPC proxies were defined that were all SNPs close to promising SNPs (distance <500 kb), in high LD (LD>0.9) and available in more than 70% of the individuals of the second stage. Results of the second stage analyses underwent the same quality control as first stage results. Combined analyses The combined analyses of all first and second stage GWAS was performed with METAL [35] with inverse variance based method. Results for men and women were combined as described for the first stage meta-analyses. All promising loci for which at least one proxy had a genome-wide significant P value in the combined analysis were named genome-wide significant loci and the best SNP of the combined analyses (largest absolute beta) was reported as topSNP of this locus. Novel loci - conditional analyses and look-ups in previous GIANT analyses Two analyses were performed to distinguish between genome-wide significant body shape loci that are known from previous GWAS on BMI, height and WHR and novel body shape loci. First, conditional analyses were performed. We used the 226 reported topSNPs (32 BMI, 180 height, 14 WHR) of published GIANT analyses on BMI, height and WHR [1] , [2] , [4] to perform conditional analyses of the first stage meta-analyses using GCTA [15] , [48] . The results of this analysis were then analysed conditioned on 843 topSNPs (97 BMI, 697 height, 49 WHR) of the published GIANT analyses [1] , [2] , [4] . To identify the overlap of the results for AvPCs with the single anthropometric traits, the same conditional analyses were performed for BMI, height and WHR separately. For calculation of the LD-structure genotype data from KORA F4 was used. Two topSNPs of the unpublished GIANT results had to be removed before analyses as they were in high correlation with two other topSNPs. If the body shape topSNPs were independent loci identified by previous GIANT analyses, the P value should stay promising ( P value<5 × 10 −6 ) in both conditional analyses. Second, we checked by look-ups if those genome-wide significant SNPs that are independent from the previously reported topSNPs were not genome-wide significant ( P value>5 × 10 −8 ) in GIANT analyses [1] , [2] , [4] . Genome-wide significant SNPs are named novel SNPs if they fulfil the following conditions: P value of conditioned analyses on topSNPs reported by previous GIANT analyses (on BMI, height, WHR) remained promising ( P value<5 × 10 −6 ). P value in previous GIANT analyses (on BMI, height, WHR) was not genome-wide significant ( P value>5 × 10 −8 ). Pleiotropic effects For identification of potential pleiotropic effects several look-ups in various large-scale consortia on different phenotypes were performed, including GIANT, DIAGRAM and MAGIC, all references are given in the results table of the look-ups ( Supplementary Table 7 ). For comparison of effect directions the loadings of each AvPC have to be considered. For example AvPC2 includes height with a positive loading and BMI with a negative loading. That means an increasing effect on AvPC2 means an increasing effect on height but a decreasing effect on BMI. Further Analyses PCA, further analyses and plots were generated with R ( http://www.r-project.org/ ) if not stated otherwise. Apart from the GCTA analyses, which uses LD structure of KORA F4, all LD analyses were performed in PLINK based on HapMap 2 (CEU) genotypes. For comparison of findings between loci from different AvPCs two loci are assumed to be identical if the topSNPs are in high LD (LD>0.8). Data availability Summary statistics of all analyses can be downloaded from: https://www.broadinstitute.org/collaboration/giant/ How to cite this article : Ried, J. S. et al. A principal component meta-analysis on multiple anthropometric traits identifies novel loci for body shape. Nat. Commun. 7 , 13357 doi: 10.1038/ncomms13357 (2016). Publisher's note: Springer Nature remains neutral with regard to jurisdictional claims in published maps and institutional affiliations.